The seco-iridoid pathway fromCatharanthus roseus The (seco)iridoids and their derivatives, the monoterpenoid indole alkaloids (MIAs), form two large families of plant-derived bioactive compounds with a wide spectrum of high-value pharmacological and insect-repellent activities. Vinblastine and vincristine, MIAs used as anticancer drugs, are produced by Catharanthus roseus in extremely low levels, leading to high market prices and poor availability. Their biotechnological production is hampered by the fragmentary knowledge of their biosynthesis. Here we report the discovery of the last four missing steps of the (seco)iridoid biosynthesis pathway. Expression of the eight genes encoding this pathway, together with two genes boosting precursor formation and two downstream alkaloid biosynthesis genes, in an alternative plant host, allows the heterologous production of the complex MIA strictosidine. This confirms the functionality of all enzymes of the pathway and highlights their utility for synthetic biology programmes towards a sustainable biotechnological production of valuable (seco)iridoids and alkaloids with pharmaceutical and agricultural applications. Monoterpenoid indole alkaloids (MIAs) are a large group of plant-derived natural products with a range of pharmacological properties. Examples of MIAs are camptothecin—used to treat cancer—and quinine—the antimalarial drug of choice till the mid of the last century. Madagascar periwinkle, Catharanthus roseus , the best-characterized MIA-producing plant species, is the source of the valuable MIAs vincristine and vinblastine, which are used directly or as derivatives for the treatment of several cancer types. Owing to the extremely low concentrations (0.0002% fresh weight), production of vincristine and vinblastine is expensive and availability of the drug is sensitive to environmental and political instability in the production countries. Therefore, biotechnology-based production of MIAs in microorganisms or alternative plant hosts has been proposed as a sustainable substitute; however, progress has been hampered by the lack of knowledge of the enzymes responsible for MIA biosynthesis, particularly in the secologanin pathway ( Fig. 1 ). Secologanin is the monoterpenoid (also called iridoid or secoiridoid) branch end point and is coupled to tryptamine by strictosidine synthase (STR) to form strictosidine, the universal MIA precursor in plants. The secologanin pathway has broad importance as many plant species accumulate iridoids and secoiridoids (including secologanin) as end products without incorporating them into complex alkaloids. Many (seco)iridoids are bioactive themselves, with among others anticancer, antimicrobial and anti-inflammatory activities [1] , [2] , [3] , [4] . Iridoids are also pheromones in some insect species, and as such can be employed for pest management in agriculture and the control of insect-related disease vectors [5] , [6] . 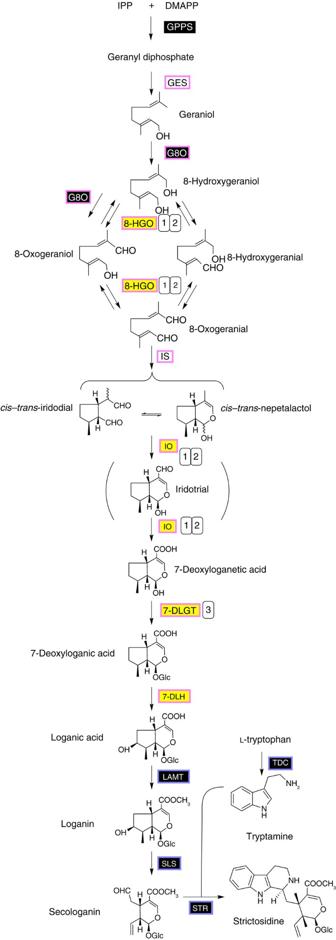Figure 1: The secologanin–strictosidine pathway. Genes indicated in boxes were published before (black background) or during (white background) the present study, or are reported here (yellow background). Frames indicate mRNA localization in the leaf IPAP (pink) or epidermis (blue). Numbers indicate predicted enzyme classes in the initial gene discovery strategy. 1: oxidoreductase, 2: cytochrome P450, 3: UGT. IPP, isopentenyl pyrophosphate; DMAPP, dimethylallyl pyrophosphate; Glc, glucose; GPPS, geranyl diphosphate synthase, GES, geraniol synthase; G8O, geraniol 8-oxidase; 8-HGO, 8-hydroxygeraniol oxidoreductase; IS, iridoid synthase; IO, iridoid oxidase; 7-DLGT, 7-deoxyloganetic acid glucosyl transferase; 7-DLH, 7-deoxyloganic acid hydroxylase; LAMT, loganic acidO-methyltransferase; SLS, secologanin synthase; STR, strictosidine synthase; TDC, tryptophan decarboxylase. Iridotrial indicated in brackets was a previously proposed intermediate that we did not detectin vitroorin vivo. Figure 1: The secologanin–strictosidine pathway. Genes indicated in boxes were published before (black background) or during (white background) the present study, or are reported here (yellow background). Frames indicate mRNA localization in the leaf IPAP (pink) or epidermis (blue). Numbers indicate predicted enzyme classes in the initial gene discovery strategy. 1: oxidoreductase, 2: cytochrome P450, 3: UGT. IPP, isopentenyl pyrophosphate; DMAPP, dimethylallyl pyrophosphate; Glc, glucose; GPPS, geranyl diphosphate synthase, GES, geraniol synthase; G8O, geraniol 8-oxidase; 8-HGO, 8-hydroxygeraniol oxidoreductase; IS, iridoid synthase; IO, iridoid oxidase; 7-DLGT, 7-deoxyloganetic acid glucosyl transferase; 7-DLH, 7-deoxyloganic acid hydroxylase; LAMT, loganic acid O -methyltransferase; SLS, secologanin synthase; STR, strictosidine synthase; TDC, tryptophan decarboxylase. Iridotrial indicated in brackets was a previously proposed intermediate that we did not detect in vitro or in vivo . Full size image The (seco)iridoid pathway is still largely unresolved. It starts with geraniol and is thought to comprise ~10 enzymes catalysing successive oxidation, reduction, glycosylation and methylation reactions ( Fig. 1 ). Although the pathway has been investigated for decades [7] , [8] , only the first step (geraniol 10-hydroxylase/8-oxidase, G8O) [9] and the two last steps (loganic acid O -methyltransferase, LAMT; and secologanin synthase, SLS) [10] , [11] are well established. Only recently, two additional enzymes were identified, iridoid synthase (IS) responsible for the reductive cyclization step [12] and geraniol synthase (GES) [13] . A complicating factor for gene discovery as well as biotechnological production is that the MIA pathway in C. roseus is organized in a complex manner, with the enzymes localized in different cell types and subcellular compartments ( Supplementary Fig. 1 ) [14] , [15] . Here we report the characterization of the last missing steps of the C. roseus secoiridoid pathway. We use an integrated transcriptomics and proteomics approach for gene discovery, followed by biochemical characterization of the isolated candidates. Furthermore, we reconstitute the entire MIA pathway up to strictosidine in the plant host Nicotiana benthamiana , by heterologous expression of the newly identified genes in combination with the previously known biosynthesis genes. This work provides essential tools that will allow development of synthetic biology platforms for the production of bioactive iridoids, secoiridoids and complex MIAs with a wide range of agricultural and pharmaceutical applications, including the treatment of cancer. Iridoid gene discovery We previously reported the assembly of CathaCyc, a C. roseus metabolic pathway database based on Illumina HiSeq2000 RNA sequencing data [16] . The data set was derived from C. roseus suspension cells and shoots treated with the plant hormone methyl jasmonate [16] . Here we complemented this data set with RNA-Seq data from cell suspensions overexpressing either ORCA2 or ORCA3 , transcription factors that regulate the expression of LAMT , SLS and several other genes in the MIA biosynthesis pathway [17] , but not GES and G8O ( Fig. 2a ). These four and all other known MIA genes are induced by MeJA both in cell suspension cultures and whole C. roseus plants, although GES/G8O and LAMT/SLS show different induction characteristics ( Fig. 2b ). Furthermore, GES , G8O and IS are expressed in the internal phloem-associated parenchyma (IPAP) cells, whereas LAMT and SLS are expressed in the leaf epidermis [10] , [11] , [12] , [13] , [18] , [19] . The differential induction and in situ expression data suggested that the first part of the pathway (possibly up to 7-deoxyloganic acid) corresponds to one transcriptional regulon, whereas the subsequent steps up to the synthesis of secologanin would comprise a second regulon. 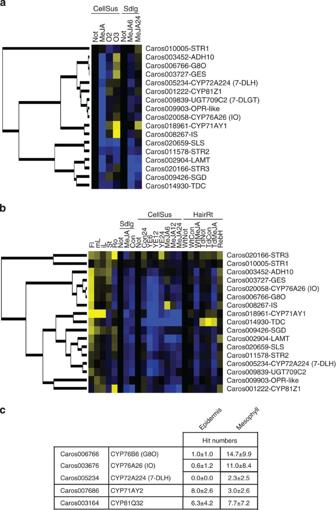Figure 2: Gene discovery strategy. (a,b) Complete-linkage hierarchical clustering of early MIA pathway gene expression inC. roseusbased on our data (a) or the Medicinal Plant Genomics Resource consortium (http://medicinalplantgenomics.msu.edu) (b). Colours indicate transcriptional activation (blue) or repression (yellow) relative to untreated samples. Tissues: Fl, flower; mL, mature leaves; iL, immature leaves; St, stem; Ro, root; Sdlg, seedling. Suspension cells (CellSus): Wt, wild-type; O2, ORCA2; O3, ORCA3. Hairy roots (HairRt): Wt, wild-type; Td, TDCi; RebH, RebH_F. Treatments: Not, no treatment; MeJA, methyl jasmonate (6, 12 or 24 h); Con, mock; YE, yeast extract. (c) Candidate P450 protein hits in the epidermis and mesophyll samples from proteomics analysis±s.d. (n=3). GES, geraniol synthase; G8O, geraniol 8-oxidase; 8-HGO, 8-hydroxygeraniol oxidoreductase; IS, iridoid synthase; IO, iridoid oxidase; 7-DLGT, 7-deoxyloganetic acid glucosyl transferase; 7-DLH, 7-deoxyloganic acid hydroxylase; LAMT, loganic acidO-methyltransferase; SGD, strictosidine β-D-glucosidase; SLS, secologanin synthase; STR, strictosidine synthase (1–3: three related genes); TDC, tryptophan decarboxylase. Figure 2: Gene discovery strategy. ( a , b ) Complete-linkage hierarchical clustering of early MIA pathway gene expression in C. roseus based on our data ( a ) or the Medicinal Plant Genomics Resource consortium ( http://medicinalplantgenomics.msu.edu ) ( b ). Colours indicate transcriptional activation (blue) or repression (yellow) relative to untreated samples. Tissues: Fl, flower; mL, mature leaves; iL, immature leaves; St, stem; Ro, root; Sdlg, seedling. Suspension cells (CellSus): Wt, wild-type; O2, ORCA2; O3, ORCA3. Hairy roots (HairRt): Wt, wild-type; Td, TDCi; RebH, RebH_F. Treatments: Not, no treatment; MeJA, methyl jasmonate (6, 12 or 24 h); Con, mock; YE, yeast extract. ( c ) Candidate P450 protein hits in the epidermis and mesophyll samples from proteomics analysis±s.d. ( n =3). GES, geraniol synthase; G8O, geraniol 8-oxidase; 8-HGO, 8-hydroxygeraniol oxidoreductase; IS, iridoid synthase; IO, iridoid oxidase; 7-DLGT, 7-deoxyloganetic acid glucosyl transferase; 7-DLH, 7-deoxyloganic acid hydroxylase; LAMT, loganic acid O -methyltransferase; SGD, strictosidine β-D-glucosidase; SLS, secologanin synthase; STR, strictosidine synthase (1–3: three related genes); TDC, tryptophan decarboxylase. Full size image On the basis of the hypothetical pathway and predicted enzyme activities catalysing the hitherto missing steps ( Fig. 1 ), we screened our data set for genes encoding NAD(P)-binding Rossmann fold domain-type oxidoreductases, cytochrome P450 monooxygenases (P450s) and UDP-glycosyltransferases (UGTs) that display co-expression with GES/G8O, and for P450s that show co-expression with LAMT/SLS . Three genes encoding putative oxidoreductases showed a high degree of co-expression with GES/G8O ( Fig. 2a ). The first (accession number Caros008267 in the ORCAE database: http://bioinformatics.psb.ugent.be/orcae [16] ) was annotated as a progesterone reductase, the second (Caros003452) as an aldehyde dehydrogenase and the third (Caros009903) as a 12-oxophytodienoate reductase. We also identified four P450s (Caros020058, Caros001222, Caros018961 and Caros005234) and one UGT (Caros009839) that showed close co-expression with GES/G8O ( Fig. 2a ). The first oxidoreductase (Caros008267) was found to encode the recently described iridoid synthase [12] , thus confirming the validity of our screening strategy. The others were selected for further functional analysis. We also verified the co-expression of these candidate genes in the publicly available data set from the Medicinal Plant Genomics Resource consortium ( http://medicinalplantgenomics.msu.edu ), which has been integrated into the ORCAE website ( http://bioinformatics.psb.ugent.be/orcae [16] ). This analysis strongly supported our selection of candidate genes ( Fig. 2b ). The tissue localization of the enzymes in the leaf was used as a second criterion to pinpoint the most promising candidate genes. This was investigated using proteomics on epidermal and mesophyll protoplasts isolated from C. roseus leaves. The proteomics analysis resulted in the identification of 2,200 proteins. Three P450s (Caros005234, Caros006766 and Caros020058) and one UGT (Caros020739) were enriched in the mesophyll fraction, whereas one P450 (Caros007986), one UGT (Caros004449) and nine oxidoreductases (Caros022489, Caros002459, Caros017236, Caros002170, Caros012730, Caros006689, Caros007544, Caros021570 and Caros003491) were enriched in the epidermal fraction. One P450 (Caros003164) was present in both tissues ( Fig. 2c and Supplementary Table 1 ). Caros003452 is the missing 8-hydroxygeraniol oxidoreductase The three oxidoreductases (Caros008267, Caros003452 and Caros009903) were produced in Escherichia coli and purified for in vitro enzyme assays. Confirming a previous report [12] , the putative progesterone reductase (Caros008267) was shown to possess IS activity in the presence of 8-oxogeranial, yielding a mixture of cis-trans -iridodial and cis-trans -nepetalactol. Caros003452 was active with the substrates 8-OH-geraniol, 8-OH-geranial and 8-oxogeraniol in the presence of NAD + , yielding mixtures of the three compounds and 8-oxogeranial in varying relative amounts depending on the combination and the incubation time ( Fig. 3 ). The enzyme was therefore coined 8-hydroxygeraniol oxidoreductase (8-HGO). With the cofactor NAD + it did not convert 8-oxogeranial ( Fig. 3 ), and it was not active with any of the substrates listed above in the presence of NADP + /NADPH. Relatively high activity was observed with some other primary alcohols such as geraniol ( Supplementary Table 2 ). Given the complex kinetics, with four interconvertible compounds and eight possible reactions, the reaction constants could not be determined. 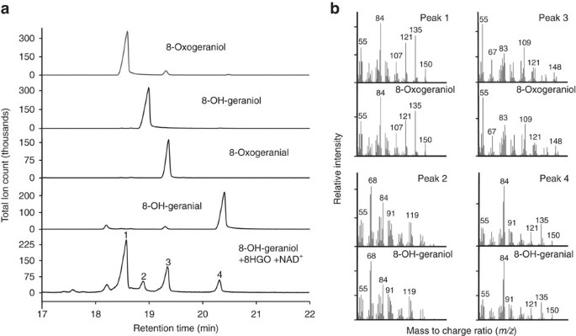Figure 3: Functional characterization of recombinant 8-HGO. Affinity-purified enzyme expressed inE. coliwas incubated with 8-OH-geraniol and NAD+. (a) GC–MS profile of the reaction extract compared with authentic standards. (b) The identity of peaks 1–4 was confirmed by comparison of MS spectra with authentic standards. 8-HGO catalyses the stepwise conversion of 8-OH-geraniol into 8-oxogeraniol or 8-OH-geranial and then into 8-oxogeranial. Figure 3: Functional characterization of recombinant 8-HGO. Affinity-purified enzyme expressed in E. coli was incubated with 8-OH-geraniol and NAD + . ( a ) GC–MS profile of the reaction extract compared with authentic standards. ( b ) The identity of peaks 1–4 was confirmed by comparison of MS spectra with authentic standards. 8-HGO catalyses the stepwise conversion of 8-OH-geraniol into 8-oxogeraniol or 8-OH-geranial and then into 8-oxogeranial. Full size image CYP76A26 is the missing iridoid oxidase Six candidate P450 genes ( CYP76A26, CYP81Z1, CYP81Q32, CYP72A224 , CYP71AY1 and CYP71AY2 ) were transferred to a yeast expression vector and co-expressed in Saccharomyces cerevisiae together with the P450 reductase ATR1 from Arabidopsis thaliana [20] ( Supplementary Fig. 2 ). Functional screening was carried out as described [21] with geraniol, 8-hydroxygeraniol, 8-hydroxygeranial, 8-oxogeraniol, 8-oxogeranial, iridodial, iridotrial, 7-deoxyloganic acid and 7-deoxyloganetic acid as potential substrates. CYP76A26 converted both iridodial and iridotrial into 7-deoxyloganetic acid. The cis- iridodial and trans- iridodial freely interconverted with cis-trans -nepetalactol [12] , and although CYP76A26 seemed to use the bicyclic nepetalactol as the preferred substrate, the monocyclic cis- and trans -iridodials were also utilized, possibly after spontaneous conversion into nepetalactol ( Fig. 4 ). The interconversion and sequential metabolism of nepetalactol and the iridodials in aqueous solution prevented reliable evaluation of the catalytic parameters with these substrates. Iridotrial was previously proposed as an intermediate of the secologanin pathway [8] . Whereas we never detected iridotrial as an intermediate in the iridodial to 7-deoxyloganetic acid conversion under conditions more likely to capture early reaction products such as low substrate concentrations, short incubations or low temperature, the latter was very efficiently converted into 7-deoxyloganetic acid with a K mapp of 25 μM and k cat of 5.2 s −1 ( Supplementary Fig. 3 ). This suggests that CYP76A26 is a multifunctional P450 enzyme catalysing successive hydroxylation/dehydration steps via a mechanism similar to that recently described for CYP701A3, which catalyses the conversion of kaurene to kaurenoic acid in the biosynthesis of gibberellins [22] . 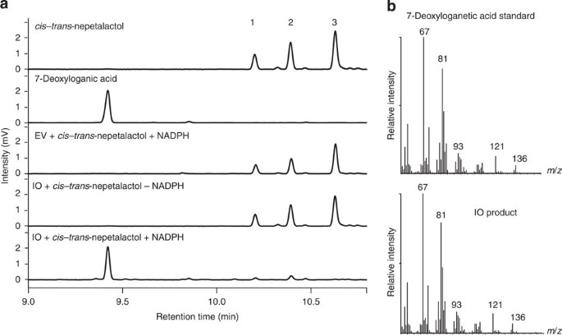Figure 4: Functional characterization of IO. The cytochrome P450 enzyme was expressed in yeast and assayed as a microsomal preparation by incubation withcis-trans-nepetalactol and NADPH. (a) GC–MS profile of the reaction extract compared with the negative control and authentic standards. (b) Product identity was confirmed by comparison of the MS spectrum with the authentic standard.Cis-trans-nepetalactol is the peak 3 (ref.13), in the substrate standard, peaks 1 and 2 are its open dialdehyde forms (cisandtransiridodial). These compounds are in equilibrium in water12. Peak 3 is the first converted by IO, but eventually, possibly after interconversion, all three compounds are metabolized (not shown). Figure 4: Functional characterization of IO. The cytochrome P450 enzyme was expressed in yeast and assayed as a microsomal preparation by incubation with cis-trans -nepetalactol and NADPH. ( a ) GC–MS profile of the reaction extract compared with the negative control and authentic standards. ( b ) Product identity was confirmed by comparison of the MS spectrum with the authentic standard. Cis-trans -nepetalactol is the peak 3 (ref. 13 ), in the substrate standard, peaks 1 and 2 are its open dialdehyde forms ( cis and trans iridodial). These compounds are in equilibrium in water [12] . Peak 3 is the first converted by IO, but eventually, possibly after interconversion, all three compounds are metabolized (not shown). Full size image As the related G8O (CYP76B6) was previously shown to oxidize several (other) monoterpene alcohols in addition to geraniol [9] , these compounds were also tested as potential substrates for CYP76A26. The enzyme converted 8-oxogeraniol into an unidentified product ( Supplementary Fig. 4 ), albeit with a low efficiency, and catalysed the hydroxylation of linalool, nerol, citronellol and lavandulol, but not geraniol ( Supplementary Fig. 4 ; Supplementary Table 3 ). CYP76A26 thus catalyses the conversion of iridodial into 7-deoxyloganetic acid and was consequently named iridoid oxidase (IO; Fig. 1 ). UGT709C2 is 7-deoxyloganetic acid glucosyl transferase The UGT (Caros009839 or UGT709C2), produced in E. coli , catalysed the glucosylation of 7-deoxyloganetic acid to form 7-deoxyloganic acid using UDP-glucose as the sugar donor ( Fig. 5 ). The enzyme had a K mapp of 9.8 μM and a k cat of 1.25 s −1 ( Supplementary Fig. 5 ). The enzyme was inactive with loganetic acid, loganetin, iridodial, iridotrial, 8-OH-geraniol, jasmonic acid, gibberellic acid, indole acetic acid, salicylic acid, abscisic acid, zeatin and luteolin. It thus behaved as a selective 7-deoxyloganetic acid glucosyl transferase (7-DLGT; Fig. 1 ). 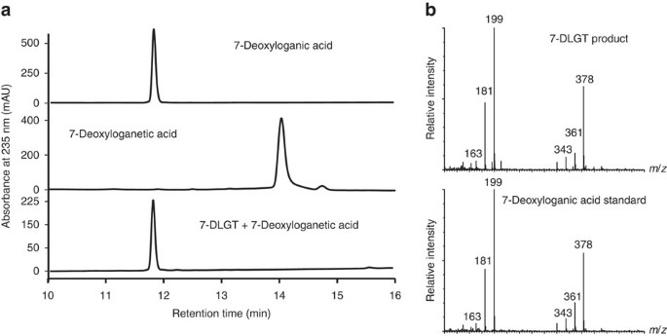Figure 5:Functional characterization of 7-DLGT. Affinity-purified enzyme expressed inE. coliwas incubated with 7-deoxyloganetic acid and UDP-glucose. (a) HPLC-DAD profile of the reaction extract compared with authentic standards. (b) Product identity was confirmed by comparison of the mass spectrum with the authentic standard. Figure 5: Functional characterization of 7-DLGT . Affinity-purified enzyme expressed in E. coli was incubated with 7-deoxyloganetic acid and UDP-glucose. ( a ) HPLC-DAD profile of the reaction extract compared with authentic standards. ( b ) Product identity was confirmed by comparison of the mass spectrum with the authentic standard. Full size image CYP72A224 is the 7-deoxyloganic acid hydroxylase Despite its poor expression in yeast, CYP72A224 catalysed the conversion of 7-deoxyloganic acid into loganic acid in yeast microsomes ( Fig. 6 ) with a K mapp of 400 μM and a V max of 0.01 pmol s −1 per mg microsomal protein ( Supplementary Fig. 6 ). k cat could not be determined due to low expression in yeast preventing precise quantification of the enzyme concentration. Owing to the low expression of CYP72A224 in yeast, a N. benthamiana leaf-disc assay was also carried out to further confirm its role in loganic acid formation ( Supplementary Fig. 7 ). The aglycone derivative of 7-deoxyloganic acid (7-deoxyloganetic acid) was not a substrate for CYP72A224, confirming that glycosylation precedes hydroxylation of the cyclopentane ring. CYP72A224 was thus named 7-deoxyloganic acid hydroxylase (7-DLH). 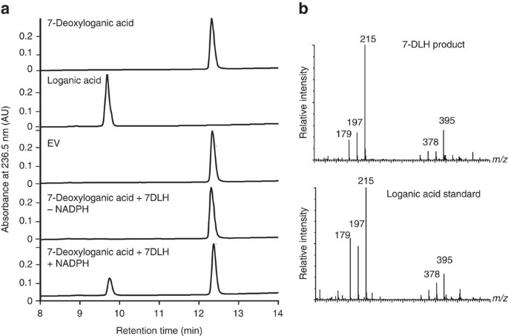Figure 6: Functional characterization of 7-DLH. The cytochrome P450 enzyme was expressed in yeast and assayed as a microsomal preparation by incubation with 7-deoxyloganic acid and NADPH. (a) HPLC-DAD profile of the reaction extract compared with the negative control and authentic standards. (b) Product identity was confirmed by comparison of the mass spectrum with the authentic standard. Figure 6: Functional characterization of 7-DLH. The cytochrome P450 enzyme was expressed in yeast and assayed as a microsomal preparation by incubation with 7-deoxyloganic acid and NADPH. ( a ) HPLC-DAD profile of the reaction extract compared with the negative control and authentic standards. ( b ) Product identity was confirmed by comparison of the mass spectrum with the authentic standard. Full size image CYP72A224 belongs to the same P450 subfamily as secologanin synthase (SLS; CYP72A1), which catalyses the conversion of loganin into secologanin [10] . Both of these P450s use glycosylated substrates and have similar regiospecificities, suggesting that SLS evolved from 7-DLH thus extending the iridoid pathway to the secoiridoids. The overlap in their substrate specificities was therefore investigated ( Supplementary Fig. 8 ). As SLS showed no 7-DLH activity and vice versa , our proposed evolutionary process appears to have yielded specific and mutually exclusive catalytic activities for each enzyme. Tissue-specific and subcellular localization of the pathway Efficient pathway engineering requires precise knowledge of the cellular and subcellular organization of different pathway components. IO, 7-DLH, 8-HGO and 7-DLGT were therefore expressed as green fluorescent protein fusions in C. roseus cells together with mCherry markers for nucleus, cytosol, endoplasmic reticulum (ER), plastids, mitochondria or peroxisomes. This revealed that IO and 7-DLH are ER-associated as predicted, whereas 8-HGO and 7-DLGT are soluble proteins found in the cytosol and the nucleus ( Supplementary Fig. 9 ). Previous in situ transcript analysis [18] , [19] , [23] suggested that a pathway intermediate is translocated from IPAP cells (the site of the early biosynthetic steps) to the epidermis, where the final steps of the pathway occur . In situ hybridization showed that 8-HGO, IO, 7-DLGT and 7-DLH are expressed in the same tissue as G8O ( Fig. 7 ). The separate clustering of the expression of these genes ( Fig. 2a ) and the similar tissue-specific transcript localization suggest that these genes constitute a transcriptional regulon for the production of loganic acid in IPAP cells. The epidermis-specific positive control SGD confirms the localization of the next transcriptional regulon, consisting of LAMT, SLS, STR and TDC , in the epidermis. The existence of this regulon is supported by the highly similar co-expression profiles of these genes as shown in Fig. 2a . 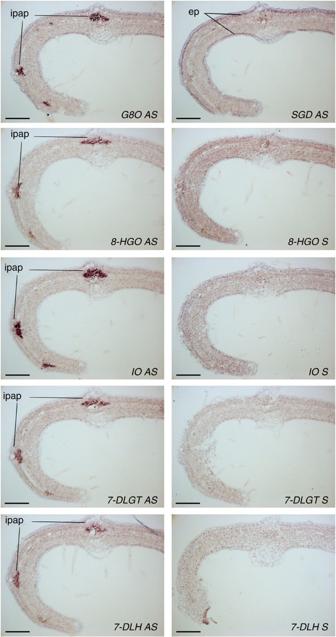Figure 7: Expression of the transcriptional regulon required for loganic acid biosynthesis in the IPAP cells. In situhybridization on serial longitudinal sections of young developing leaves was carried out with antisense (AS) probes and sense (S) probes as controls.G8Oand strictosidine β-D-glucosidase (SGD) AS probes were used as IPAP and epidermis markers, respectively. Sense probe controls gave no signals (not shown). 8-HGO, 8-hydroxygeraniol oxidoreductase; IO, iridoid oxidase; 7-DLGT, 7-deoxyloganetic acid glucosyl transferase; 7-DLH, 7-deoxyloganic acid hydroxylase; IPAP, internal phloem-associated parenchyma; ep, epidermis. Scale bar=100 μm. Figure 7: Expression of the transcriptional regulon required for loganic acid biosynthesis in the IPAP cells. In situ hybridization on serial longitudinal sections of young developing leaves was carried out with antisense (AS) probes and sense (S) probes as controls. G8O and strictosidine β-D-glucosidase ( SGD ) AS probes were used as IPAP and epidermis markers, respectively. Sense probe controls gave no signals (not shown). 8-HGO, 8-hydroxygeraniol oxidoreductase; IO, iridoid oxidase; 7-DLGT, 7-deoxyloganetic acid glucosyl transferase; 7-DLH, 7-deoxyloganic acid hydroxylase; IPAP, internal phloem-associated parenchyma; ep, epidermis. Scale bar=100 μm. Full size image Reconstitution of strictosidine synthesis in N. benthamiana The identification of the four enzymes described above allowed us to propose a complete secologanin pathway ( Fig. 1 ), which we tested by stepwise combinatorial transient expression of the corresponding genes in N. benthamiana ( Fig. 8 ). To boost substrate availability for the pathway, a geranyl diphosphate synthase from Picea abies ( PaGPPS ) [24] and a geraniol synthase from Valeriana officinalis ( VoGES) [25] were used because the C. roseus orthologues were not available at the onset of these studies. The transient expression of PaGPPS+VoGES in N. benthamiana resulted in the formation of geraniol, but also several additional oxidized and glycosylated derivatives were detected, presumably produced by endogenous N. benthamiana enzymes as previously reported [25] . The stepwise addition of G8O and IS resulted in the generation of new compounds, including new derivatives of the anticipated pathway intermediates (combinations 1, 2 and 4 in Fig. 8a,b ; Supplementary Fig. 10 ). In contrast, the addition of 8-HGO to the combination PaGPPS+VoGES+G8O only modified the existing product profile quantitatively but did not generate any new compounds (combination 3 in Fig. 8a,b ; Supplementary Fig. 10 ). This is probably due to the fact that endogenous N. benthamiana enzymes have similar activity as 8-HGO ( Supplementary Fig. 11 ). When IO was co-expressed with PaGPPS+VoGES+G8O+8-HGO+IS (combination 5), the metabolic profile did not change, and 7-deoxyloganetic acid and its derivatives were not detected ( Fig. 8a,b ). 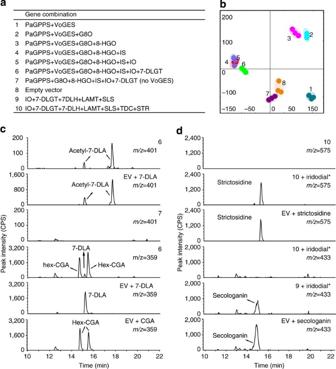Figure 8:Reconstitution of the strictosidine pathway inN. benthamiana. (a) Gene combinations infiltrated in leaves in triplicate. (b) Principal component analysis. PC1 and PC2 describe 36.2 and 31.1% of the total mass variation, respectively. (c) LC-MS analysis showing selected masses 401 and 359 representing (acetylated) 7-deoxyloganic acid (7-DLA) from infiltrations with 8-carboxygeranic acid (CGA), 7-DLA or gene combinations 6 or 7 (negative control). The two peaks likely represent 7-DLA acetylated at two different positions in the glucose moiety. (d) LC-MS analysis showing selected masses 433 (formic acid adduct of secologanin) and 575 (formic acid adduct of strictosidine) from infiltrations with secologanin or strictosidine, or with gene combinations 9 or 10, with or without iridodial. *Identical profiles with iridotrial or 7-DLH. Hex=hexosyl; CPS=counts per second. However, reconstitution of the pathway up to 7-DLGT (combination 6) was successful and resulted in the production of 7-deoxyloganic acid and putative acetylated 7-deoxyloganic acid ( Fig 8a,c ). Without IO , these products were not detected ( Supplementary Fig. 12 ), indicating that IO is functional in N. benthamiana and is an essential part of the biosynthesis pathway. These findings also illustrate the importance of full pathway coverage for functional analysis of individual enzymes. Figure 8: Reconstitution of the strictosidine pathway in N. benthamiana. ( a ) Gene combinations infiltrated in leaves in triplicate. ( b ) Principal component analysis. PC1 and PC2 describe 36.2 and 31.1% of the total mass variation, respectively. ( c ) LC-MS analysis showing selected masses 401 and 359 representing (acetylated) 7-deoxyloganic acid (7-DLA) from infiltrations with 8-carboxygeranic acid (CGA), 7-DLA or gene combinations 6 or 7 (negative control). The two peaks likely represent 7-DLA acetylated at two different positions in the glucose moiety. ( d ) LC-MS analysis showing selected masses 433 (formic acid adduct of secologanin) and 575 (formic acid adduct of strictosidine) from infiltrations with secologanin or strictosidine, or with gene combinations 9 or 10, with or without iridodial. *Identical profiles with iridotrial or 7-DLH. Hex=hexosyl; CPS=counts per second. Full size image Subsequently, the entire postulated secologanin pathway ( PaGPPS to SLS) was introduced by agroinfiltration; however, this only yielded products up to 7-deoxyloganic acid. Therefore, we increased the input halfway into the pathway by infiltrating the intermediates iridodial, iridotrial or 7-deoxyloganic acid in combination with the pathway genes. In all cases this resulted in the production of secologanin, indicating that the second half of the pathway is also functional ( Fig. 8d ). When 7-DLH, LAMT or SLS were omitted from combination 9—with infiltration of the intermediates iridodial, iridotrial or 7-deoxyloganic acid—no secologanin was detected showing that all conversions require the infiltrated C. roseus genes ( Supplementary Fig. 13 ). Finally, we tested whether the biosynthesis pathway up to secologanin can be functionally combined with the tryptamine branch of the MIA pathway. When the secologanin biosynthesis pathway genes were co-infiltrated with the tryptophan decarboxylase ( TDC ) and STR genes, and the flux through the pathway was boosted by co-infiltration of the intermediates iridodial, iridotrial or 7-deoxyloganic acid, strictosidine was indeed produced (combination 10 in Fig. 8d ). Whereas feeding experiments clearly indicated that secologanin is derived from geraniol [26] , the exact sequence of intermediates and enzymes leading to the formation of its penultimate precursor loganic acid was still obscure. We report here four novel enzymes that together with two previously reported enzymes [12] , [13] fill the existing gaps and thereby provide a full description of the core (seco)iridoid pathway. Geraniol is converted to secologanin by the sequential action of four different cytochrome P450 enzymes, two different oxidoreductases, one glucosyltransferase and one methyltransferase. The missing enzymes and corresponding genes were identified by a combination of transcriptomic and proteomic approaches exploiting the current knowledge of the spatiotemporal regulation of the secoiridoid pathway. Our results also address longstanding questions in the field. First, as previously proposed for oxidoreductase proteins purified from Rauwolfia serpentina and Nepeta racemosa [27] , [28] , 8-HGO catalyses two successive and reversible oxidation steps for the formation of 8-oxogeranial. Therefore, two enzymes can contribute to the formation of the intermediate 8-oxogeraniol. G8O was recently shown to also produce 8-oxogeraniol from geraniol [21] , thus G8O and 8-HGO appear to catalyse partially overlapping (and in the case of G8O, monodirectional) oxidation reactions that result in the production of 8-oxogeraniol from 8-hydroxygeraniol ( Fig. 1 ). Second, a single cytochrome P450 enzyme IO/CYP76A26 can convert cis-trans -iridodial and cis-trans -nepetalactol into 7-deoxyloganetic acid without the release of an iridotrial intermediate. Third, our data demonstrate that 7-deoxyloganetic acid glycosylation precedes its further oxygenation by 7-DLH. This answers the longstanding question which intermediate is transferred from IPAP cells to the epidermis. The expression of 7-DLH in IPAP cells indicates that loganic acid is the mobile intermediate transferred to the epidermis, and hence that glycosylation by 7-DLGT is not sufficient for mobility but that further hydroxylation by 7-DLH is also required. The tissue-specific expression of pathway sections may increase the flux through the pathway by alleviating feedback inhibition by intermediates and products, and/or it may segregate the iridoid and secoiridoid/MIA pathways, allowing them to fulfill tissue-specific functions. Pathway reconstitution experiments in a heterologous host validated the enzyme sequence leading to the formation of strictosidine ( Fig. 1 ). We however observed a low flux through the pathway in the leaves of N. benthamiana . Previous experiments carried out with the upstream segment of the pathway indicated substantial conversion of intermediate products to other oxidized, acetylated, malonylated and glycosylated derivatives by endogenous N. benthamiana enzymes [21] . Despite downstream channeling of intermediates upon reconstruction of the full pathway, competing conversions are still observed and are probably responsible for the low flux. This would, for example, explain why we cannot see the product of IO upon infiltration of pathway combination 5 ( Fig. 8 ; Supplementary Fig. 12 ). Nevertheless, we know that IO is functional because infiltration of combination 9 or 10 with iridodial did result in production of secologanin or strictosidine, respectively ( Fig. 8d ). Side reactions could possibly be eliminated by further metabolic engineering. The side products obtained in our experiments may also provide valuable information on the enzyme networks naturally present in N. benthamiana and could be leads for combinatorial biochemistry programmes to produce chemical diversity and novel bioactive compounds. In conclusion, we have identified the four missing enzymes in the secologanin pathway in C. roseus . In combination with the genes previously identified, the genes encoding these four enzymes are sufficient to engineer secologanin production and, together with TDC and STR , biosynthesis of the complex alkaloid strictosidine in the heterologous plant N. benthamiana . Although different segments of the strictosidine pathway are localized in different cell types in C. roseus , our results show that the entire pathway can be successfully reconstituted in a single N. benthamiana organ. This paves the way for the biotechnological production of valuable (seco)iridoids and derived compounds, such as the MIAs vincristine and vinblastine, making these important anticancer drugs available to more people and at a lower price. Chemicals The substrates 8-carboxygeranial, 8-carboxygeranic acid, 8-oxogeranic acid and 8-hydroxygeranic acid were synthesized on order by Synthelor (Vandoeuvre-Lès-Nancy, France), whereas 8-OH-geraniol, 8-oxogeraniol, 8-OH-geranial and 8-oxogeranial were synthesized by Chiralix B.V. (Nijmegen, Netherlands). Iridodial-glucoside, iridotrial-glucoside and 7-deoxyloganic acid were synthesized from aucubin extracted from Aucuba japonica leaves by Chiralix B.V. as described [29] , [30] . The aglucone iridoid pathway intermediates were produced by incubation with almond β-glucosidase (Sigma-Aldrich) in 50 mM acetate buffer (pH 5). Loganetic acid and loganetin were produced by the deglucosylation of loganic acid and loganin (Extrasynthese). Aglycones were extracted with diethyl ether, evaporated under N 2 and quantified by 1 H-NMR ( 1 H-nuclear magnetic resonance). Transcriptomic analysis Transgenic derivatives of C. roseus cell line MP183L (overexpressing the ORCA transcription factors) were generated by particle bombardment [31] with derivatives of the pER8 plasmid [32] carrying either the ORCA2 or ORCA3 open reading frames (ORFs). Selected transgenic lines were treated for 24 h with 10 μM estradiol, and RNA was isolated as described [16] . Illumina HiSeq2000 RNA sequencing, assembly, annotation and mapping of the RNA-Seq reads on the reference transcriptome was carried out as described [16] . Complete linkage hierarchical cluster analysis was achieved using the CLUSTER and TREEVIEW software [33] and the log 10 transformed values of the normalized FPKM values were used as input for CLUSTER. Proteomic analysis For the plant material of C. roseus var. little Bright Eyes seeds were sown in sterilized soil and covered with transparent plastic until germination. The soil was kept humid. The plants were fertilized weekly with 0.2% liquid Wuxal (29 g l −1 nitrate-N; 46 g l −1 ammonium-N; 25 g l −1 carbamide-N; 100 g l −1 P 2 O 5 total phosphate; 75 g l −1 K 2 O; 124 mg l −1 B; 50 mg l −1 Cu; 248 mg l −1 Fe; Cu, Fe, Mn and Zn as EDTA-chelate). The plants were re-potted twice during further growth. For the isolation of epidermal protoplasts, y oung, light-green C. roseus leaves (length 4–7 cm) from side branches (without buds or flowers) of 8- to 11-week-old plants were harvested for protoplast isolation. The mid-vein was removed and the leaves were cut into 1- to 2-mm strips. Protoplasts were isolated as described [34] . To collect epidermal protoplasts, a layer of 1-ml betaine solution (0.5 M betaine, 1 mM CaCl 2 , 10 mM MES, pH 5.6 with KOH) was added on top of the tubes containing the protoplast mix. After centrifugation for 7 min at 1,500 r.p.m. and 4 °C, epidermal protoplasts were collected from the upper interphase. The suspension was mixed with 4-ml protoplast solution and 25% Percoll (pH 6), and overlaid with 1.5 ml of betaine solution for a second purification step. The tubes were centrifuged at 700 r.p.m. for 30 min and the epidermal protoplasts were again collected from the upper interphase. Protoplasts were pelleted in the betaine solution. Isolation of mesophyll protoplasts was performed as described for the epidermal protoplasts with replacement of the MCP solution with TEX solution (3.2 g l −1 Gamborg’s B5 medium, 3.1 mM NH 4 NO 3 , 5.1 mM CaCl 2 , 2.6 mM MES, 0.4 M sucrose, pH 5.6–5.8 with 0.5 M KOH), and the betaine solution was replaced with mannitol/W5 (1 mM D -glucose, 30 mM NaCl, 25 mM CaCl 2 , 1 mM KCl, 0.3 mM MES, 320 mM α-mannitol, pH 5.6–5.8 with KOH). For the first gradient, 5–10% Percoll (pH 6) was added instead of 3–5%. The protoplast pellet was resuspended in 2–4 ml buffer A (20 mM HEPES pH 7.2, 1 tablet per 10 ml Roche Protease Inhibitor, 1 mM PMSF). The mixture was pressed 10–20 times through a syringe with needle and centrifuged for 10 min at 3,000 r.p.m. and 4 °C. The samples were ultra-centrifuged for 1 h at 30,000 r.p.m. The membrane pellets were dissolved in 1 ml washing solution (0.3 M NaCI, 20 mM HEPES-KOH pH 7.2, 1 tablet per 10 ml Roche Protease Inhibitor, 1 mM PMSF) by stirring with a small brush, and then vortexed for 30 s. The microsomes were frozen at –80 °C for at least 1 h, thawed and then centrifuged for 1 h at 30,000 r.p.m. and 4 °C. The pellets were dissolved in 50–100 μl buffer A for further analysis. The protein concentration was determined using the Bio-Rad DC protein assay according to the manufacturer’s instructions. For mass spectrometry analysis, ~50 μg of protein was separated by one-dimensional gel electrophoresis [35] in 10% polyacrylamide gels to reduce sample complexity. The gels were stained with Coomassie Brilliant Blue, the lanes were cut into 10 slices, the proteins were reduced with tris(carboxyethyl)phosphine hydrochloride and sulhydryl groups were blocked with iodoacetamide. In-gel digestion with sequencing-grade-modified trypsin (Promega V5111) was carried out overnight at 37 °C [36] . The resulting peptides were recovered by adding 40 mM Tris-HCl (pH 8.0) and 50% acetonitrile/1% formic acid. The peptide mixtures were desalted by solid-phase extraction on C 18 reversed-phase columns and analysed on an LTQ Orbitrap mass spectrometer (Thermo Fischer Scientific, Bremen, Germany) coupled to an Eksigent Nano HPLC system (Eksigent Technologies, Dublin, CA, USA) as previously described [37] . For protein identification, databases were searched using Mascot v2.3. Raw data were searched against a composite database consisting of all entries in the NCBI Viridiplantae database (released in November 2010), all publicly available C. roseus -expressed sequence tags (downloaded from NCBI in November 2010) and the reference transcriptome released on CathaCyc and ORCAE [16] (database contained forward and reverse protein entries, total number of protein entries 1,166,013). The parameters for precursor and fragment ion mass tolerance were set to 5 p.p.m. and 0.8 Da, respectively. One missed trypsin cleavage was allowed. Carboxyamidomethylation of cysteine was specified as fixed modification, and oxidation of methionine and pyroglutamate formation from glutamine were selected as variable modifications. Scaffold v3.0 (Proteome Software, Portland, OR, USA) was used to validate and quantify MS/MS-based peptide and protein identifications. Peptide identifications were accepted if they were established at >95% probability as specified by the Peptide Prophet algorithm [38] . Protein identifications were accepted if they were established at >90% probability and at least one peptide was uniquely assigned to a corresponding protein in a minimum of two of our samples. Protein probability was assigned by the Protein Prophet algorithm [39] . Proteins that were identified with the same set of peptides and could not be differentiated by the MS/MS analysis were grouped to protein clusters to satisfy the principles of parsimony. Peptide and protein false-discovery rates (FDR) were determined by the Scaffold software. A peptide FDR of 0.01% and a protein FDR of 0.2% were computed. The Scaffold software was also used to determine protein abundance in the mesophyll and epidermal factions based on the number of spectra assigned to each protein. An F-test was applied to assess significant differences in protein abundances. Gene isolation ORFs were amplified by PCR from a pACT2 cDNA library of a C. roseus cell culture elicited with yeast extract [40] using the primers listed in Supplementary Table 4 . For expression in plants, the ORFs were transferred to vector pRT101 (ref. 41 ) to bring them under the control of the Cauliflower Mosaic Virus 35S promoter, and the expression cassettes were then transferred to the binary vector pCAMBIA1300 (Cambia). For expression in E. coli , the ORFs were transferred to vector pASK-IBA45plus (IBA) and/or pET16-H (Novagen pET-16b derivative). Probes for in situ hybridization were prepared from the same ORFs cloned in pBluescript II SK+. For localization analysis, the ORFs were transferred to vector pTH2 (refs 42 , 43 ) and/or pTH2BN (a derivative of pTH2). The marker for nucleocytosolic localization (pRT101-mCherry) was prepared by amplifying the mCherry ORF from plasmid ER-rk [44] (The Arabidopsis Information Resources, TAIR, clone CD3-959). Isolation of His-tagged recombinant proteins Recombinant proteins carrying a His 6 tag were expressed using plasmid pASK-IBA45plus and/or pET16-H in E. coli strain BL21 (DE3) pLysS and were purified using Ni-NTA agarose chromatography (Qiagen). For quality analysis, the recombinant proteins were separated by 12.5% (w/v) SDS–PAGE, transferred to Protran nitrocellulose membranes (Whatman) by semidry electroblotting, and western blots were probed with mouse monoclonal anti-His horseradish peroxidase-conjugated antibodies (5Prime). Antibody binding was detected by incubation in 250 μM sodium luminol, 0.1 M Tris–HCl (pH 8.6), 3 mM H 2 O 2 and 67 μM p -coumaric acid, followed by exposure to an X-ray film. Enzymatic assays of UGT and oxidoreductases UGT activity was detected in 0.1-ml reaction buffer containing 50 mM potassium phosphate (pH 7.5), 2 mM UDP-glucose, 5–1,000 μM 7-deoxyloganetic acid or 2 mM of other tested compounds and 50–1,000 ng of purified enzyme. Reactions were incubated at 32 °C for 15 min and stopped by adding 1 volume of methanol, mixed by vortexing and kept on ice for 10 min. The tubes were centrifuged at 4,000 g for 10 min, and the supernatants were passed through 0.22-μm nylon filters. Oxidoreductase activity was detected in 1-ml reaction buffer containing 50 mM bis-tris propane (pH 9 for oxidation and pH 7.5 for reduction), 2–1,000 μM 8-OH-geraniol, 8-oxogeraniol, 8-OH-geranial, 8-oxogeranial or other tested compounds, 2–2,000 μM NAD + or NADH and 50–1,000 ng of purified enzyme. Reactions were incubated for 15 min at 32 °C, stopped by adding 0.2 volumes of 1 M sodium citrate (pH 3) and centrifuged and filtered as above. Quantitative assays were carried out by measuring NADH production at 340 nm in a Nanodrop2000c (Thermoscientific) Chromatographic analysis of 8-HGO and 7-DLGT products Identification of 8-HGO enzyme products was performed using capillary gas chromatography mass spectrometry. The ethyl acetate extract of the reaction mixture was separated on a Agilent GC 7890A series equipped with a 5975C MSD and DB-5 capillary column (30 m × 0.25 mm, film thickness of 0.25 μm; JpW Scientific). Helium gas was used as a carrier at a flow rate of 1.2 ml min −1 . The separation conditions were as follows: split mode 1:5, injection volume 5 μl, injector temperature 230 °C, initial oven temperature 60 °C, and then linear gradient to 100 °C at a rate of 20 °C min −1 followed by a linear gradient to 160 °C at a rate of 2 °C min −1 (run time 32 min). Analysis of 7-DLGT products was carried out using an Agilent series 1200 HPLC with a diode array detector and a Polymer Laboratories PL-ELS 2100 ICE evaporative light scattering detector and a Phenomenex Luna 5 micron 150 × 4.6-mm C 18 column. The injection volume was 10 or 100 μl. The binary solvent system consisted of acetonitrile and 0.1% trifluoroacetic acid in water. The elution program was as follows: 5 min isocratic 10% acetonitrile and then 25 min gradient until 95% acetonitrile. Peak areas were calculated using Agilent ChemStation. NMR Structures of enzyme products were analysed by NMR spectroscopy in 750 μl of acetone-d 6 or methanol-d 4 in a 5-mm NMR glass tube [45] . Subcellular localization studies C. roseus MP183L cell suspension cultures were maintained by weekly 10-fold dilution in 50 ml Linsmaier & Skoog (LS) medium containing 88 mM sucrose, 2.7 μM 1-NAA and 0.23 μM kinetin (LS-13). The cells were grown at 25 °C with an 18/6-h light–dark cycle. The cells were bombarded [28] using the plasmids pTH2-IO, pTH2-7-DLH, pTH2-7-DLGT, pTH2BN-7-DLGT, pTH2-8-HGO and pTH2BN-8-HGO. The first two were combined with equal amounts of the ER marker ER-rk, and the others with the nucleocytosolic marker mCherry [44] . Bombarded cells were placed on Petri dishes with LS-13 medium and viewed after 24 h using a Zeiss Observer laser scanning microscope. In situ hybridization pBluescript plasmid derivatives containing the cDNAs for 8-HGO, IO, 7-DLGT and 7-DLH were used for the synthesis of antisense and sense digoxigenin-labelled riboprobes as previously described [19] . G8O antisense probes [19] and SGD antisense probes [46] were used as internal phloem-associated parenchyma and epidermis markers, respectively. Paraffin-embedded serial longitudinal sections of young developing leaves were hybridized with digoxigenin-labelled riboprobes and localized with antidigoxigenin-alkaline phosphatase-conjugated antibodies [47] . P450 expression in yeast and enzyme assays P450-coding sequences were amplified from pRT101 source vectors using specific primers to introduce USER sites at the ends of each sequence. The genes were subsequently transferred to the plasmid pYeDP60 using the USER cloning technique (New England Biolabs, Ipswich, UK) [48] . The resulting recombinant plasmids were introduced into S. cerevisiae strain WAT11, cultivated at 28 °C and P450 expression was induced as described [21] . Cells were harvested by centrifugation and manually broken with 0.45-mm glass beads in 50 mM Tris–HCl buffer (pH 7.5) containing 1 mM EDTA and 600 mM sorbitol. The homogenate was centrifuged for 10 min at 10,000 g and the supernatant was centrifuged for 1 h at 30,000 g . The pellet, comprising microsomal membranes, was resuspended in 50 mM Tris–HCl (pH 7.4), 1 mM EDTA and 30% (v/v) glycerol with a Potter‐Elvehjem homogenizer and stored at –20 °C. All procedures for microsomal preparation were carried out at 0–4 °C. P450 expression was evaluated as described [49] and enzymatic activities were determined in a standard 0.1 ml assay comprising for IO 2.3 nmol cytochrome P450, 0.6 mM NADPH and substrate in 20 mM sodium phosphate (pH 7.4). The reaction was initiated by the addition of NADPH and was stopped after 5 min by the addition of 10 μl 1 M HCl. Iridoids were extracted in 1 ml ethyl acetate, and the organic phase was concentrated to 200 μl before GC-FID analysis on a Varian 3900 gas chromatograph (Agilent Technologies) equipped with a flame ionization detector and a DB-5 column (30 m, 0.25 mm, 0.25 μm; Agilent Technologies) with splitless injection, at 250 °C injector temperature, and with a temperature programme of 0.5 min at 50 °C, 10 °C min −1 to 320 °C, and 5 min at 320 °C. For 7-DLH, 10 μl of yeast microsomes expressing 7-DLH (130 μg of microsomal protein) were incubated for 20 min at 27 °C, in 0.1 ml of 20 mM Na-phosphate (pH 7.4) containing 0.6 mM NADPH and substrate. The reaction was initiated by the addition of NADPH and was stopped after 20 min on ice. After addition of 50 μl of 50% acetic acid, tubes were vortexed and centrifuged. The supernatant was run on reverse-phase HPLC (Alliance 2695 Waters system, NOVA-PAK C18 4.6 × 250 mm column) with photo-diode array detection at 236.5 nm. Peak areas of the product(s) were used to calculate the catalytic parameters of each enzyme. Leaf disc assays Five-week-old N. benthamiana leaves were infiltrated with A. tumefaciens transformed with vector pCAMBIA1300 containing the relevant candidate genes, plus the helper plasmid p19. Five days post infiltration, leaves were used in a leaf disc assay as previously described [21] . Pathway reconstruction in N. benthamiana The pathway genes were transiently expressed in the leaves of five-week-old N. benthamiana plants by agroinfiltration as previously described [25] . Briefly, bacteria carrying the relevant expression constructs ( PaGPPS, VoGES, G8O, 8-HGO, IS, IO, 7-DLGT, 7-DLH, LAMT, SLS, TDC, STR, empty vector or TBSV p19 (ref. 50 )) were grown individually at 28 °C for 24 h. Cells were harvested by centrifugation and then resuspended in infiltration buffer containing 10 mM MES (Duchefa Biochemie), 10 mM MgCl 2 and 100 μM acetosyringone (4′-hydroxy-3′,5′-dimethoxyacetophenone, Sigma) to a final OD 600 of ~0.5. For all gene combinations that compared subsequent steps in the pathway, the amounts of cell suspension for each expression construct were kept constant by adding the corresponding amount of A. tumefaciens carrying an empty vector. All infiltrations were performed in three replicates. In several experiments, pathway intermediates were injected into the same leaves 3 days after agroinfiltration. Compounds used for infiltration were diluted to a final concentration of 400 μM in methanol/water (1:19), with the same ratio of methanol/water alone as a negative control and 400 μM 7-deoxyloganic acid, 8-carboxygeranic acid, secologanin or strictosidine as positive controls. Leaves were harvested for metabolite analysis 5 days after agroinfiltration. Frozen, powdered N. benthamiana leaves (200 mg aliquots) were extracted in 0.6 ml 99.867% methanol, 0.133% formic acid and 5 μl of the extract was analysed using a Waters Alliance 2795 HPLC connected to a QTOF Ultima V4.00.00 mass spectrometer (Waters, MS Technologies, UK). Measurements were taken in negative ionization mode. LC-MS data were acquired using MassLynx 4.0 (Waters) and processed using MetAlign version 1.0. The normalized and log-transformed data matrix was used for principal component analysis implemented in GeneMath XT v 2.1. ANOVA was used to evaluate the statistical significance of differences in metabolite levels between all treatments. How to cite this article: Miettinen, K. et al . The seco-iridoid pathway from Catharanthus roseus . Nat. Commun. 5:3606 doi: 10.1038/ncomms4606 (2014). Accession Codes: Transcriptomic data have been deposited in the GenBank Sequence Read Archive (SRA) under the accession code SRP026417 . Gene sequences have been deposited in GenBank nucleotide core database under the accession codes KF302066 (IO), KF302067 (7DLH), KF302068 (7DLGT), KF302069 (8-HGO), KF302070 (CYP81Q32), KF302071 (CYP81C13), KF302072 (CYP71AY2), KF302073 (CYP71BT1), KF302074 (CYP72A225), KF302075 (CYP76T24), KF302076 (CYP71D2), KF302077 (ADH9), KF302078 (ADH13), KF302079 (ADH14), KF302080 (UGT9) and KF309243 (CYP71AY1).